In situliquid-cell electron microscopy of silver–palladium galvanic replacement reactions on silver nanoparticles Galvanic replacement reactions provide an elegant way of transforming solid nanoparticles into complex hollow morphologies. Conventionally, galvanic replacement is studied by stopping the reaction at different stages and characterizing the products ex situ . In situ observations by liquid-cell electron microscopy can provide insight into mechanisms, rates and possible modifications of galvanic replacement reactions in the native solution environment. Here we use liquid-cell electron microscopy to investigate galvanic replacement reactions between silver nanoparticle templates and aqueous palladium salt solutions. Our in situ observations follow the transformation of the silver nanoparticles into hollow silver–palladium nanostructures. While the silver–palladium nanocages have morphologies similar to those obtained in ex situ control experiments the reaction rates are much higher, indicating that the electron beam strongly affects the galvanic-type process in the liquid-cell. By using scavengers added to the aqueous solution we identify the role of radicals generated via radiolysis by high-energy electrons in modifying galvanic reactions. Solution synthesis has demonstrated unprecedented control over the size, shape and morphology of nanoparticles of different metals. Furthermore, initially homogeneous metal nanoparticles with well-defined shapes can serve as a starting material in galvanic replacement reactions, in which they are used as sacrificial templates to produce hollow and porous nanostructures with complex morphologies, such as nanoboxes or nanocages [1] , [2] , [3] , [4] , [5] , [6] , [7] , [8] , [9] . Such hollow and porous structures have drawn interest as they can shift plasmon resonances compared with those of solid nanoparticles [5] , [10] , may provide nanoscale containers for biomedical applications such as diagnostics and drug delivery [11] , are of use as contrast enhancement agents in optical imaging such as optical coherence [12] , photoacoustic tomography [13] , [14] , and are found to be highly active in catalysis [15] , [16] , [17] , [18] , [19] , [20] and electrocatalysis [21] , [22] . The galvanic replacement reaction is critical in the advanced two-step synthesis of fuel cell electrocatalysts with reduced precious metal loadings, limited to a thin surface layer or even a monolayer on top of less expensive metal nanoparticles [23] , [24] , [25] , [26] , [27] , [28] , [29] , [30] , [31] , [32] , [33] . The electrocatalysts obtained either via the transmetalation of an underpotentially deposited [23] , [26] , [28] or electrodeposited [27] , [29] , [30] , [31] , [32] , [33] monolayer or thin layer of a less precious metal by a precious metal upon immersion into a complex solution of Pt, Pd or Au ions [23] , [26] , [27] , [28] , [29] , [30] , [31] , [32] , [33] , or by partial galvanic replacement [24] , [25] exhibit enhanced activity compared to the most active Pt catalysts [23] , [24] , [25] , [26] , [27] , [28] , [29] , [30] , [31] , [32] , [33] . Galvanic replacement reactions using Ag nanoparticles as sacrificial templates have recently been demonstrated as a simple and elegant way of producing hollow and porous nanostructures of noble metals (Au, Pd and Pt) [3] , [6] , [8] . When a suspension of Ag nanoparticles is titrated with aqueous solutions of different metal precursors, such as HAuCl 4 or PdCl 2 , galvanic replacement between the two species occurs spontaneously and leads to the formation of hollow nanoparticles whose morphology depends on that of the starting templates. In the reaction, [AuCl 4 ] − or [PdCl 4 ] 2− oxidizes Ag to AgCl, which causes the hollowing-out of the sacrificial Ag templates. The morphological and structural changes of nanoparticles due to galvanic replacement are typically investigated ex situ by transmission electron microscopy (TEM) on samples taken at different stages of the reaction [34] . So far, the only in situ observation of the process on the nanoscale has been a transmission X-ray microscopy study of galvanic replacement in large (>100 nm diameter) Ag nanowires with 10–15 nm spatial resolution [35] . In situ closed-cell microscopy, capable of imaging processes in liquid environments enclosed between thin SiN membranes in real time by TEM or scanning TEM (STEM), has the potential to go beyond this ‘quench-and-look’ approach and image reactions while they occur in solution. Liquid-cell microscopy has made considerable progress recently. It provides a platform for the quantitative analysis of nanoparticle dynamics in liquids, of solution growth without [36] , [37] or with [38] , [39] a template, and of electrochemical deposition [40] , [41] , [42] , and has been shown to be capable of sub-nanometer resolution [43] , [44] . Nanoparticle growth within the liquid cell is generally initiated through reduction of a precursor by the imaging electron beam [36] , [37] , [39] , [45] , [46] , [47] , though decoupling the growth from electron beam effects has been explored [37] . Nanoparticle dynamics observed within the liquid cell generally deviate from Brownian motion due to electron beam effects and interactions with the enclosing SiN membranes, facilitating the continuous imaging of individual nanostructures in solution [48] , [49] . While in situ observations can provide unique insight into processes in liquid environments, the imaging electron beam invariably affects these processes, for example, by creating radicals such as hydrated electrons that can reduce metal salts and thus drive or accelerate redox chemistry. To properly interpret liquid-cell experiments and to be able to use electron irradiation judiciously to control in situ solution chemistry, it is important to understand the effects caused by the electron beam. Here we use liquid-cell TEM and STEM to investigate galvanic replacement reactions and their modification by radicals generated via radiolysis by a high-energy electron beam. Specifically, we consider reactions in Pd-salt solutions, which transform Ag nanoparticle templates into complex Ag–Pd nanostructures. Real-time observations allow us to follow the evolution of Ag templates into porous and solid nanocages, to directly identify the role of the electron beam in this process and to gain insight into novel pathways for modifying galvanic replacement processes. To study galvanic-type reactions and the effects of high-energy electron irradiation, we perform complementary experiments comprising real-time in situ liquid-cell TEM and STEM, as well as control experiments in which reactions are set to proceed on the bench without electron irradiation. In both cases, ex situ electron microscopy and complementary analytical methods are used to evaluate the reaction products with high spatial resolution and chemical specificity. Galvanic replacement without electron irradiation Before discussing the results of in situ (S)TEM experiments, we establish the behaviour observed via the conventional ‘quench-and-look’ approach, in which the reaction—proceeding in absence of an electron beam (that is, on the bench)—is stopped at defined intervals and the resulting morphologies are imaged by TEM and STEM. These data provide a benchmark for determining modifications induced by the electron beam during in situ observations of the reaction. We focus on a replacement reaction involving the oxidation of Ag nanoparticles and reduction of Pd ions in an aqueous PdCl 2 solution generally used for electrochemical Pd deposition on different substrates [39] . The prevailing Pd complexes in the aqueous solution are metal–chloro complexes, that is, tetrachloropalladate ions (PdCl 4 ) 2− , which are reduced by the capture of two electrons: (PdCl 4 ) 2− +2e − ⇌ Pd+4Cl − . Figures 1a,b and 2a,b show TEM and high-angle annular dark-field (HAADF) STEM images of the starting Ag nanoparticles, respectively. The majority of the Ag particles are multiple twinned ( Figs 1b and 2b ), often with irregular shapes comprising several corners and asperities. The majority of the particles have diameters between 29 and 33 nm; the mean diameter is 31.2±0.25 nm ( Fig. 2c ). 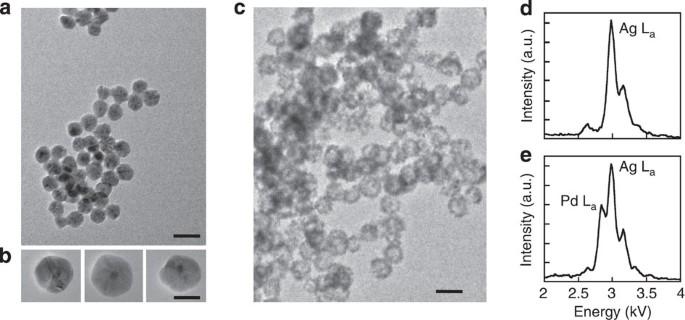Figure 1: Galvanic replacement of Ag particles in Pd-salt solution without electron irradiation. (a) TEM image of the initial Ag nanoparticles; scale bar, 50 nm. (b) HR-TEM images of three representative Ag nanoparticles; scale bar, 20 nm. (c) TEM image of the Ag–Pd hollow nanostructures formed after 4 h of immersion of the Ag nanoparticles in 50 μM PdCl2aqueous solution. For ease of comparison, the image scale is identical to that ina; scale bar, 50 nm. (d,e) EDS spectra of a Ag nanoparticle and a Ag–Pd hollow-shell nanostructure, respectively. Figure 1: Galvanic replacement of Ag particles in Pd-salt solution without electron irradiation. ( a ) TEM image of the initial Ag nanoparticles; scale bar, 50 nm. ( b ) HR-TEM images of three representative Ag nanoparticles; scale bar, 20 nm. ( c ) TEM image of the Ag–Pd hollow nanostructures formed after 4 h of immersion of the Ag nanoparticles in 50 μM PdCl 2 aqueous solution. For ease of comparison, the image scale is identical to that in a ; scale bar, 50 nm. ( d , e ) EDS spectra of a Ag nanoparticle and a Ag–Pd hollow-shell nanostructure, respectively. 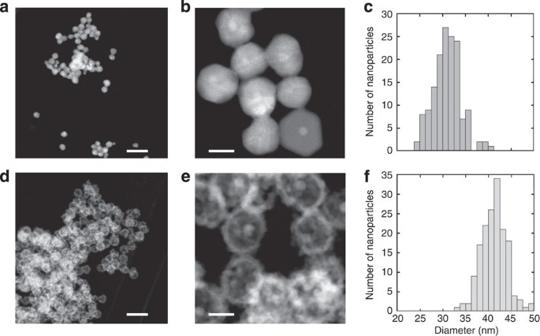Figure 2: Morphology and size distribution changes of Ag nanoparticles during galvanic replacement in Pd-salt solution without electron irradiation. HAADF–STEM images of (a,b)—the initial Ag nanoparticles and (d,e) the Ag–Pd hollow nanostructures formed after 4 h of immersion of the Ag nanoparticles in 50 μM PdCl2aqueous solution. To facilitate comparison, the image scales are identical ina,d, (scale bar, 100 nm) and inb,e(scale bar, 20 nm). Distribution of nanoparticle sizes of (c)—the initial Ag nanoparticles and (f)—the Ag–Pd nanostructures. Full size image Figure 2: Morphology and size distribution changes of Ag nanoparticles during galvanic replacement in Pd-salt solution without electron irradiation. HAADF–STEM images of ( a , b )—the initial Ag nanoparticles and ( d , e ) the Ag–Pd hollow nanostructures formed after 4 h of immersion of the Ag nanoparticles in 50 μM PdCl 2 aqueous solution. To facilitate comparison, the image scales are identical in a , d , (scale bar, 100 nm) and in b , e (scale bar, 20 nm). Distribution of nanoparticle sizes of ( c )—the initial Ag nanoparticles and ( f )—the Ag–Pd nanostructures. Full size image The reaction of Ag particles in a 50 μM PdCl 2 precursor solution (see Methods for details) was carried out at room temperature to ensure conditions identical to those in the microscope. Imaging of the nanoparticles at different stages, that is, by quenching the reaction after 1, 2 and 4 h after immersion in the Pd solution showed the development of characteristic morphological and chemical changes. The nanoparticles hollowed out gradually, that is, transformed into porous crystalline shells ( Figs 1c and 2d,e ). The hollowing of the nanoparticles was accompanied by a distinct increase in size. The particle size distribution shifted significantly towards larger sizes, and after 4 h, the majority of the nanoparticles have diameters between 36 and 44 nm; the mean diameter is 41.2±2.2 nm ( Fig. 2f ). Energy-dispersive X-ray spectroscopy (EDS) analysis ( Fig. 1e ) shows that the shells contain both Ag and Pd, with high Ag content (~65–70 at. % Ag). We further attempted to determine the elements exposed in the outermost atomic layer by low-energy ion scattering spectroscopy (ISS). These measurements were not conclusive due to the similar mass of Ag and Pd atoms ( Supplementary Fig. 1 ). Instead, X-ray photoelectron spectroscopy (XPS) of both Ag and Pd core levels, and especially of Pd Auger transitions, provided clear evidence of the composition and chemical state of Pd and Ag in the hollow nanoshells. Both investigations were performed on nanoparticle ensembles identical to the ones shown in Figs 1c and 2d , dispersed on Ge substrates. XPS on the Ag–Pd nanoshells confirms the presence of Ag ( Fig. 3a ) and Pd ( Fig. 3c ). The Ag 3d 5/2 peak (~368.15 eV) is shifted to lower binding energy compared with a Ag single crystal reference (~368.3 eV, Fig. 3b ), in agreement with a similar shift observed upon alloy formation in small Ag–Pd clusters and Ag and Pd supported clusters [50] . The Pd 3d 5/2 peak (~335.1 eV) is not significantly shifted from the reported value for pure Pd single crystals. However, a significant shift would not be expected since upon alloying with up to 50% Ag, the Pd 3d 5/2 binding energy shifts by at most 0.1 eV, that is, it is insensitive to alloying with Ag in this concentration range [50] . The Pd M 4,5 VV Auger spectrum is more suitable to detect alloying with Ag, as it has characteristic fine structure that changes with alloying, that is, can be used to quantify the composition of Ag–Pd alloys [50] , [51] , [52] . The line shape of the Pd M 4,5 VV Auger spectrum measured on our Ag–Pd nanoshells ( Fig. 3d ) indicates that Pd is in a Ag 0.7 Pd 0.3 alloy, that is, the measurement confirms the formation of a Ag–Pd alloy upon formation of the hollow nanoshells. 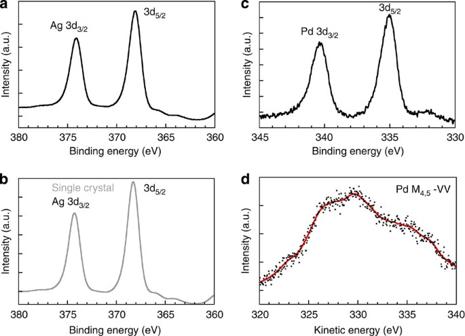Figure 3: X-ray photoelectron spectroscopy of the Ag–Pd hollow shell nanostructures. (a) X-ray photoelectron spectra of Ag 3d core levels of the composite Ag–Pd nanoshells compared with (b) the Ag 3d spectra of a silver single crystal standard. (c) X-ray photoelectron spectrum of Pd 3d core levels of the nanoshells. (d) Pd Auger electron spectrum of the composite Ag–Pd nanoshells formed by galvanic replacement. Figure 3: X-ray photoelectron spectroscopy of the Ag–Pd hollow shell nanostructures. ( a ) X-ray photoelectron spectra of Ag 3d core levels of the composite Ag–Pd nanoshells compared with ( b ) the Ag 3d spectra of a silver single crystal standard. ( c ) X-ray photoelectron spectrum of Pd 3d core levels of the nanoshells. ( d ) Pd Auger electron spectrum of the composite Ag–Pd nanoshells formed by galvanic replacement. Full size image Longer reaction times did not lead to significant further changes in morphology. The Pd content stayed at a maximum of ~30–35 at. %, similar to earlier results on galvanic replacement reactions between these two metals [3] . The Pd content could not be increased further, neither by increasing the Pd-salt concentration in the solution (up to 1 mM) nor the reaction time. Previous work for the Pd–Ag system showed a termination of galvanic replacement once nanoboxes composed of a Pd–Ag alloy containing~30–35 at. % Pd was produced, suggesting that the formation of a homogeneous alloy (or possibly coverage by a complete Pd monolayer) eliminated the electrochemical driving force for the further oxidation of Ag [53] . This is unlike Au–Ag [1] , [3] , where a much larger difference in the standard electrochemical potentials drives the galvanic replacement beyond the nanobox stage and a complete de-alloying can be achieved [3] , [34] . Real-time TEM imaging of galvanic-type reactions Ag nanoparticles were introduced in PdCl 2 aqueous solution identical to those used in our benchtop reference experiments, loaded into the liquid cell and subjected to in situ TEM and STEM observations of the galvanic replacement process. 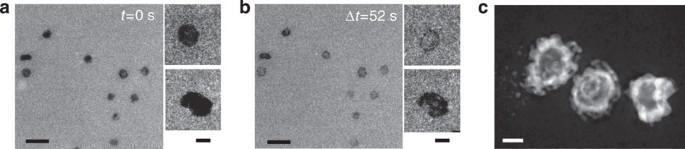Figure 4:Evolution of Ag particles in 10 μM aqueous PdCl2solution duringin situTEM imaging. (a) Initial TEM image of an ensemble of Ag nanoparticles in the liquid cell (scale bar, 100 nm) and higher magnification images of two of the particles (right of panel, scale bar, 20 nm). (b) The same group of nanoparticles (scale bar, 100 nm), and the same two individual particles (right of panel, scale bar 20 nm) after 52 s. Electron dose rate: 15.6 e−Å−2s−1. Total dose per image: 5.2 e−Å−2. Cumulative electron dose betweenaandb: 811 e−Å−2. (c)Ex situhigh-resolution Z-contrast image of three Ag–Pd nanoparticles formed in the process (scale bar. 20 nm). Figure 4 shows representative in situ TEM observations of Ag nanoparticles in PdCl 2 aqueous solution (see also Supplementary Movie 1 ). Figure 4a is an initial TEM image of a group of Ag nanoparticles. While Ag particles in aqueous solution without PdCl 2 are generally imaged with homogenous contrast, the particles in the PdCl 2 solution are slightly hollow already in the initial image, due to the fact that a galvanic replacement reaction starts at the moment of immersing the particles in the solution, about 10–15 min before the first images are obtained in the microscope. Following the further evolution of the particle morphology over time, we find that the particles lose contrast very quickly as the Ag in their interior is depleted and holes develop in their surface. Figure 4b shows in situ liquid TEM images of the same group of particles after 52 s elapsed observation time. The particles now appear completely hollowed out, that is, have transformed into empty shells. Z-contrast images ( Figs 4c and 5 ) taken after quenching the reaction and opening the liquid cell confirm that the particles are empty porous shells with homogenous composition. The cages are Ag rich and contain 10–20 at. % Pd, as shown by EDS ( Supplementary Fig. 2 ). The highest Pd content we detected in a survey of several Ag–Pd nanocages was ~20 at. %. Finally, Z-contrast images (for example, Fig. 5b ) show that the porous nanocages are invariably surrounded by numerous small Ag-containing nanoparticles. Figure 4: Evolution of Ag particles in 10 μM aqueous PdCl 2 solution during in situ TEM imaging. ( a ) Initial TEM image of an ensemble of Ag nanoparticles in the liquid cell (scale bar, 100 nm) and higher magnification images of two of the particles (right of panel, scale bar, 20 nm). ( b ) The same group of nanoparticles (scale bar, 100 nm), and the same two individual particles (right of panel, scale bar 20 nm) after 52 s. Electron dose rate: 15.6 e − Å −2 s −1 . Total dose per image: 5.2 e − Å −2 . Cumulative electron dose between a and b : 811 e − Å −2 . ( c ) Ex situ high-resolution Z-contrast image of three Ag–Pd nanoparticles formed in the process (scale bar. 20 nm). 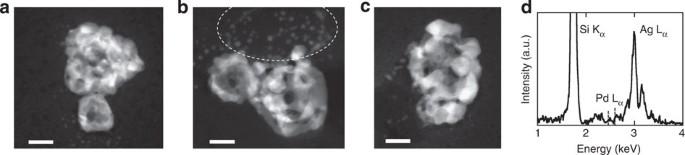Figure 5:Ex situcharacterization of Ag–Pd nanocages formed duringin situTEM observations. (a–c) High-resolution HAADF–STEM images of representative porous Ag–Pd nanocages; scale bar, 20 nm. Note the arrays of small nanoparticles in the vicinity of the larger nanocages (outlined by a dashed oval). (d) EDS spectrum from a Ag–Pd nanocage. Full size image Figure 5: Ex situ characterization of Ag–Pd nanocages formed during in situ TEM observations. ( a – c ) High-resolution HAADF–STEM images of representative porous Ag–Pd nanocages; scale bar, 20 nm. Note the arrays of small nanoparticles in the vicinity of the larger nanocages (outlined by a dashed oval). ( d ) EDS spectrum from a Ag–Pd nanocage. Full size image Ex situ high-resolution bright-field STEM and HAADF–STEM ( Fig. 6a,b , respectively) of the larger Ag–Pd nanocage in Fig. 5b , shows that the shells are crystalline and that holes have formed in the crystalline matrix. Tilt series ( Supplementary Movie 2 ) demonstrate that the holes are distributed over the entire surface, that is, the shells are porous single crystalline nanocages. 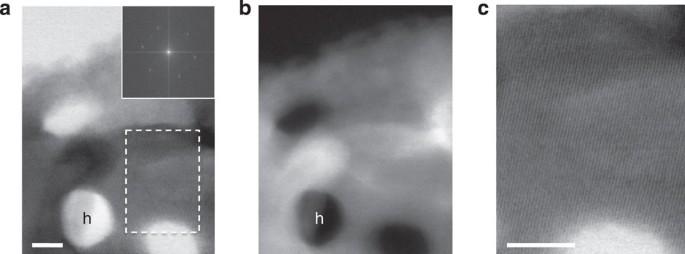Figure 6: High-resolution imaging of Ag–Pd nanocages. (a,b) High-resolution BF-STEM and HAADF–STEM images of a representative hollow cage Ag–Pd nanoparticle (inset: FFT of the entire nanocage,Fig. 5b). h, hole in the nanoparticle surface. Scale bar, 5 nm. (c) Higher magnification of the square area marked ina. Scale bar, 5 nm. Figure 6: High-resolution imaging of Ag–Pd nanocages. ( a , b ) High-resolution BF-STEM and HAADF–STEM images of a representative hollow cage Ag–Pd nanoparticle (inset: FFT of the entire nanocage, Fig. 5b ). h, hole in the nanoparticle surface. Scale bar, 5 nm. ( c ) Higher magnification of the square area marked in a . Scale bar, 5 nm. Full size image The comparison of the in situ observations of Ag nanoparticles in aqueous PdCl 2 solution with the results of the galvanic displacement reaction in the same solution on the bench shows several close similarities. In both cases, there is a transformation from nanoparticles to nanocages, accompanied by an overall size increase to diameters of ~40 nm similar to the one observed in the galvanic experiments on the bench. Occasionally, larger particles of ~65 nm are also observed, likely generated by coalescence of closely spaced smaller Ag nanoparticles ( Fig. 4a ). Hence, we conclude that the reaction observed in situ in the liquid cell is also a redox process. However, the hollowing-out of the Ag particles and conversion into porous Ag–Pd nanocages occurs much faster than in the benchtop galvanic replacement reaction. This difference in the reaction rates suggests that the electron beam strongly affects the galvanic-type process in the liquid cell. In situ observations show a significant loss of Ag in the particle interior during the initial 8 s of observation, that is, within this brief interval the Ag particles undergo changes that require ~2 h on the bench. The fact that the fast replacement reaction is localized within the field-of-view (FOV) in TEM further supports our conclusion that the electron beam plays an important role in driving the reaction in the liquid cell, that is, represents an invasive probe that alters the reaction rate, and possibly the reaction pathway as well. Real-time STEM imaging of galvanic-type reactions The way in which electrons are delivered in the two imaging modes, TEM and STEM, is very different [46] . In TEM, the FOV is exposed uniformly and at constant rate to a collimated electron beam, whereas in STEM a tightly focused beam is scanned across the FOV and delivers high electron doses during brief time intervals into sub-nanometer spots within the liquid cell. To gain additional information on the role of the electron beam in galvanic processes in aqueous solution, we performed in situ experiments in STEM mode. 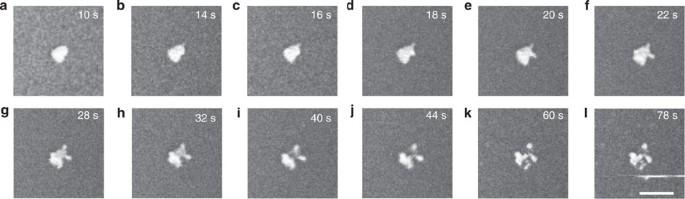Figure 7:Evolution of Ag particles in 10 μM aqueous PdCl2solution duringin situSTEM imaging. (a–l) Sequence of HAADF–STEM images following the evolution of a Ag particle in 10 μM aqueous PdCl2solution. Electron dose rate: 48 e−Å−2s−1; frame time: 2.1 s. Electron dose per image: 102 e−Å−2. Scale bar, 100 nm. Figure 7 shows a series of dark-field STEM images tracking the evolution of a characteristic Ag nanoparticle in the aqueous PdCl 2 solution (10 μM PdCl 2 ). The Ag particles are very mobile (for example, Supplementary Movies 3 and 4 ) and with each time-step the number of the nanoparticles in the FOV changes due to sudden displacements (‘jumps’) [39] , [54] . In Figs 7a–l and 8a–f , we track individual particles that could reliably be followed as they remain in the FOV during the entire sequence. Figure 7: Evolution of Ag particles in 10 μM aqueous PdCl 2 solution during in situ STEM imaging. ( a – l ) Sequence of HAADF–STEM images following the evolution of a Ag particle in 10 μM aqueous PdCl 2 solution. Electron dose rate: 48 e − Å −2 s −1 ; frame time: 2.1 s. Electron dose per image: 102 e − Å −2 . Scale bar, 100 nm. 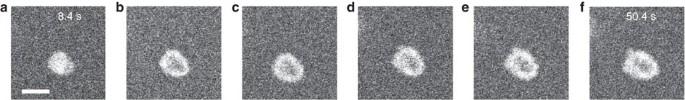Figure 8:Evolution of a representative Ag particle in 50 μM aqueous PdCl2solution. (a–f): Time-lapse series of dark-field STEM images following one Ag particle over 50.4 s in 50 μM aqueous PdCl2solution. Electron dose rate: 6.26 e−Å−2s−1, frame time: 8.4 s. Electron dose per image: 52 e−Å−2. Scale bar, 50 nm. Full size image Figure 8: Evolution of a representative Ag particle in 50 μM aqueous PdCl 2 solution. ( a – f ): Time-lapse series of dark-field STEM images following one Ag particle over 50.4 s in 50 μM aqueous PdCl 2 solution. Electron dose rate: 6.26 e − Å −2 s −1 , frame time: 8.4 s. Electron dose per image: 52 e − Å −2 . Scale bar, 50 nm. Full size image From one frame to the next (Δ t =2.1 s), the Ag particle changes gradually in such a way that it transforms into a hollow nanostructure within 20–30 s. The particle increases in size by the deposition of Pd and formation of a Ag–Pd alloy during hollowing-out of the Ag from the particle core. Large holes develop in parallel with a pronounced thickening of corners and the Ag particle transforms into a porous hollow cage, similar to the behaviour of the Ag nanoparticles we observed during TEM imaging. The time scale of the nanoparticle-to-nanocage transformation is similar (order of seconds) independent of the imaging mode, TEM or STEM. There is a substantial difference in the morphology of the nanocages depending on the mode of observation. In contrast to the behaviour during TEM imaging—a hollowing-out similar to the replacement reaction on the bench, and complete absence of homogeneous nucleation in the solution—the cages formed in STEM grow thicker over time. Furthermore, significant homogeneous nucleation and growth in the solution surrounding the cages occurs in the whole range of electron dose rates and in the Pd precursor concentrations surveyed here (10–50 μM PdCl 2 ; 3–50 e − Å −2 s −1 ), in agreement with our earlier observations [39] . The morphology of the Ag–Pd shell nanostructures generated during in situ STEM imaging was investigated ex situ via high-resolution Z-contrast imaging ( Supplementary Fig. 2 ), which clearly shows the porous morphology of the nanocages. The concentration of Pd (up to 44 at. %) is higher than that obtained on the bench or under electron irradiation in TEM mode. The morphology of the shells can be controlled by the molarity of the Pd precursor metal complexes in the solution. In 50 μM PdCl 2, for instance, ( Fig. 8 and Supplementary Figs 3 and 4 , Supplementary Movies 3 and 4 ) large holes never develop, and a solid shell appears to thicken in consecutive image frames (8.4 s per frame). EDS maps show that Pd and Ag are uniformly distributed over the shell, with Pd content varying between 0 and 44 at. %. The overview image in Supplementary Fig. 3a shows Ag particles with large variations in the degree of transformation into Ag–Pd shells, a consequence of different times spent in the FOV and exposed to the electron beam, due to the high mobility of the Ag nanoparticles. The thickening of the shell is more pronounced for particles near the centre of the FOV where the beam resides longer, consistent with previous observations on the growth of Pd–Au core-shell nanoparticles [39] . Particles outside the FOV (that is, not irradiated by the beam) show much slower morphological changes, consistent with the rates of galvanic replacement without electron irradiation. The comparison of our ex situ experiments on the bench and of real-time electron microscopy observations in liquid cells allows us to obtain unprecedented insight into the effects of high-energy electrons on galvanic replacement reactions. In the galvanic reaction on the bench, the Ag nanoparticles undergo a slow hollowing-out, whose rate is controlled by the electrochemical potentials of the involved species. In brief, the sacrificial Ag template is oxidized by the (PdCl 4 ) 2− to Ag + , which rapidly reacts with Cl − ions to form AgCl. The electrons (e G − ) generated in the oxidation half-reaction reduce (PdCl 4 ) 2− to Pd 0 at the surface of the Ag particles. The standard reduction potential of the (PdCl 4 ) 2− /Pd pair (0.62 V versus standard hydrogen electrode (SHE)) is higher than that of the AgCl/Ag pair (0.22 V versus SHE) [3] , that is, the overall redox reaction is expected to proceed spontaneously (equation (1)): Pd and Ag have the same fcc structure, similar lattice constants and can interdiffuse at room temperature. Hence, Pd atoms incorporated in the Ag surface form small Pd–Ag alloy patches. The Ag oxidation proceeds via the formation of holes, through which Ag from the particle interior can be released into the solution over the period of a couple of hours. According to theoretical calculations and earlier experiments, the overall driving force for the galvanic displacement vanishes and the galvanic reaction stops once the hollow shell becomes a homogeneous Ag–Pd alloy [3] , [8] , [53] . High-energy electron beams affect aqueous solutions through the radiolysis of water, a process in which a number of transient species are generated. The reaction cascades induced by radiolysis can be very complex. The major species generated include hydrated electrons (e aq − )—strong reducing agents that can react with metal ions or charged complexes in solution at a diffusion-controlled rate to form zero-valent metal atoms or atom clusters [55] , [56] , [57] —and hydroxyl radicals (OH · ) [56] , which can act as potent oxidizers. The reduction by e aq − is well-established for Pd complexes, (PdCl 4 ) 2− +2e aq − ⇌ Pd 0 +4Cl − , and was used in real-time electron microscopy of the growth of Pd nanoparticles and Au–Pd core-shell nanostructures in aqueous solution [39] . The presence of beam-induced species, such as e aq − and OH · can cause major deviations from the conventional galvanic replacement reaction (equation (1)). The OH · radicals can react with one another and form H 2 O 2 , or with e aq − to form OH − , or with alcohols. At different experimental parameters, it is thus possible to achieve net oxidizing or reducing conditions, which has been exploited for a long time for preparation of nanoparticles by gamma radiolysis [58] , [59] . In contrast to the galvanic process on the bench, where the reduction of (PdCl 4 ) 2− requires e G − generated via the oxidation of Ag, the electron beam creates a second population of reducing agents, that is, e aq − generated by radiolysis. In addition to the long-lived e aq − (lifetime t ~1 μs) [39] , [60] , radiolysis by the electron beam liberates short-lived ( t ~ns), highly reactive OH · radicals [61] , [62] , [63] . Our previous observations of the Pd nanoparticle growth in liquid-cell STEM show that OH · radicals do not play a significant role in liquid-cell microscopy of Pd growth, likely due to the fact that overall reducing conditions are achieved as the hydrated electrons diffuse much further and have a longer lifetime [39] . However, the real-time observations shown here, along with control experiments discussed below, indicate that OH · radicals can be important in galvanic-type processes. Indeed, the presence of abundant OH · can explain the vastly accelerated oxidation of Ag in our liquid-cell experiments compared with the reaction on the bench. OH · enables a second redox pathway (equation (2)), which essentially decouples the oxidation of Ag from the reduction of (PdCl 4 ) 2− (that is, generation of e G − ). It is well-known that alcohols react effectively with OH · , primarily via hydrogen abstraction producing a radical and H 2 O [56] . OH · is quenched by isopropanol according to: . To support our conclusion that OH · accelerates Ag oxidation in liquid-cell microscopy, we have performed control experiments in which isopropanol was added to the aqueous PdCl 2 solution to scavenge OH · radicals. 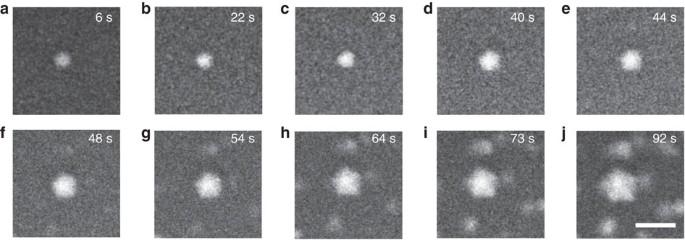Figure 9:Evolution of a representative Ag particle in 10 μM aqueous PdCl2solution with added isopropanol. (a–j) Sequence of HAADF–STEM images following the evolution of a Ag particle in 10 μM aqueous PdCl2solution with added isopropanol. Electron dose rate: 48 e−Å−2s−1; frame time: 2.1 s. Electron dose per image: 102 e−Å−2. Scale bar, 100 nm. Figure 9 shows selected images from time-lapse series of liquid-cell STEM images of the evolution of a Ag nanoparticle in 10 μM aqueous PdCl 2 , to which 0.1 mM of isopropanol were added. The hollowing-out, previously observed on the bench and in liquid-cell (S)TEM, is now completely suppressed. Instead, the particle progressively increases in size, apparently by deposition of Pd on the Ag nanoparticle core, similar to the formation of Au–Pd core-shell nanoparticles [39] . In addition, homogeneous nucleation of Pd clusters takes place in the solution. We conclude that eliminating OH · radicals from the solution without affecting the population of e aq − had the effect of dramatically lowering the Ag oxidation rate while the rate of (PdCl 4 ) 2− reduction remained high, as the CH 3 C · OHCH 3 radical is a strong reducing system (E°((CH 3 ) 2 CO/(CH 3 ) 2 C · OH)=−1.8 V) also able to reduce (PdCl 4 ) 2− , reinforcing the effect of e − aq via Figure 9: Evolution of a representative Ag particle in 10 μM aqueous PdCl 2 solution with added isopropanol. ( a – j ) Sequence of HAADF–STEM images following the evolution of a Ag particle in 10 μM aqueous PdCl 2 solution with added isopropanol. Electron dose rate: 48 e − Å −2 s −1 ; frame time: 2.1 s. Electron dose per image: 102 e − Å −2 . Scale bar, 100 nm. Full size image Overall, this shifted the reaction from a radical-modified galvanic replacement to the growth of Pd on the Ag cores, that is, formation of a Ag–Pd core-shell nanostructure. A similar shift between these reactions can also explain the different morphologies obtained in liquid-cell TEM and STEM imaging, that is, porous versus solid nanocages. The characteristics observed in STEM—higher Pd concentration in the nanocages and homogeneous nucleation of Pd particles in the surrounding solution—suggest that the focused electron beam in STEM creates more abundant e aq − , and thus enables a second pathway of Pd 0 formation (via equation (3)) that does not require e G − from the galvanic oxidation of Ag. In the extreme case of STEM imaging of Ag particles in concentrated aqueous PdCl 2 solutions, significant Ag oxidation does not take place and the Ag particles are no longer hollowing-out. Instead, rapid Pd deposition causes the formation of a core-shell structure in which a solid Ag core is surrounded by a Pd shell. In summary, by comparing the results of the in situ experiments to the ones obtained in control experiments without the influence of the electron beam we identify how solution phase redox chemistry is modified by radicals generated via radiolysis by a high-energy electron beam. We demonstrate the use of scavengers to both identify and control the radicals responsible for observed enhancements in the in situ reaction rates. In future studies such scavengers can be used judiciously to minimize electron beam effects and achieve reaction conditions close to those realized on the bench. Materials Solutions of palladium chloride (PdCl 2 , Fisher Scientific) were made by dissolving 88.65 mg of the salt in 300 μl HCl, which was then diluted with water to concentrations between 10 and 100 μM. For seeded growth, Ag nanoparticles (British Biocell International) with sizes of 20 and 30 nm and different concentrations (4.5 × 10 11 particles per ml and 1.3 × 10 11 particles per ml, respectively) were introduced in the solutions. Observations of Pd growth by liquid-cell electron microscopy were carried out at different PdCl 2 concentrations above 5 μM PdCl 2 , the threshold for observable Pd growth under the observation conditions used here. Solutions with two different concentrations were used: 10 μM PdCl 2 for STEM imaging, and 50 μM PdCl 2 for both STEM and TEM imaging of the transformations of Ag nanoparticles in solution. In situ liquid-cell TEM and STEM experiments The liquid experiments were carried out in a dedicated specimen holder (Hummingbird Scientific) using liquid cells consisting of two 30 nm thick SiN membrane windows with 50 × 50 μm 2 window area. The spacing between the windows was controlled using 90 nm polystyrene beads or 100 and 200 nm SiO 2 spacers. Bowing of the thin membrane allows a continuous range of liquid thicknesses to be established within the same cell [39] . (S)TEM imaging was performed in a FEI Titan 80–300 environmental Cs-corrected (in TEM mode) microscope operated at 300 kV. Low-loss electron energy loss spectra (EELS) were acquired on a Gatan Enfina spectrometer with an entrance aperture semiangle of 3.5 mrad. The local fluid thickness was calculated using low-loss EELS according to ref. 39 For the reaction followed in Supplementary Movie 1 and Fig. 4 the fluid thickness was ~330 nm and the electron dose per image was 5.2 e − Å −2 . STEM imaging was performed with ~2 Å beam size and beam current between 0.18 and 0.22 nA, measured in vacuum before introduction of the liquid cell. Typical conditions for the acquisition of growth series were an electron dose rate between 5 and 50 e − Å −2 s −1 and a fluid path length of 200–300 nm. Suitable serial acquisition imaging conditions were achieved by focusing at an appropriate distance from the area of interest, followed by blanking of the beam and translation to the area of interest. This procedure guaranteed that the area had not been exposed to electrons prior to scanning the first frame. A background intensity gradient visible in the images is likely related to the variation in fluid thickness. Ex situ characterization High-resolution STEM images of the Au–Pd nanostructures were acquired ex situ using a Hitachi HD2700C 200 kV cold-field emission C s -corrected STEM. X-ray photoemission spectroscopy (XPS) and low-energy ISS was carried out in a UHV system with 1 × 10 −9 Torr base pressure, equipped with a SPECS Phoibos 100 spectrometer. The XPS measurements were carried out on Ag–Pd nanoshell ensembles deposited on Ge(111) substrates and reference Ag single crystal using Mg Ka radiation. The surface composition was probed by ISS measurements using 2 keV He-ions (SPECS IQE 12/38) ion source. The analyzer was normal to the sample surface while the X-ray and ion sources were positioned 45° off the surface normal. Both electrons and ions were detected with a 5-channel electron multiplier (Specs, MCD-5) mounted on the hemispherical analyzer. How to cite this article: Sutter, E. et al. In situ liquid-cell electron microscopy of silver–palladium galvanic replacement reactions on silver nanoparticles. Nat. Commun. 5:4946 doi: 10.1038/ncomms5946 (2014).